A fast and accurate SNP detection algorithm for next-generation sequencing data Various methods have been developed for calling single-nucleotide polymorphisms from next-generation sequencing data. However, for satisfactory performance, most of these methods require expensive high-depth sequencing. Here, we propose a fast and accurate single-nucleotide polymorphism detection program that uses a binomial distribution-based algorithm and a mutation probability. We extensively assess this program on normal and cancer next-generation sequencing data from The Cancer Genome Atlas project and pooled data from the 1,000 Genomes Project. We also compare the performance of several state-of-the-art programs for single-nucleotide polymorphism calling and evaluate their pros and cons. We demonstrate that our program is a fast and highly accurate single-nucleotide polymorphism detection method, particularly when the sequence depth is low. The program can finish single-nucleotide polymorphism calling within four hours for 10-fold human genome next-generation sequencing data (30 gigabases) on a standard desktop computer. Detecting genetic variations in human genome is vital to understanding the causes of phenotypic variations, including susceptibilities to cancers and infectious diseases. Single-nucleotide polymorphisms (SNPs) are one of the most common types of genetic variation in humans. SNPs have been reported to influence protein coding [1] , transcriptional regulation [2] , alternative splicing [3] and non-coding RNA regulation [4] . A large number of SNPs has been identified in the Human Genome Project [5] , [6] and the Human Haplotype Map Project [7] , [8] . In addition, recent advances in next-generation sequencing (NGS) technologies have enabled us to detect even more SNPs. The use of NGS platforms, such as the Illumina Genome Analyzer, Roche/454 FLX and ABI SOLiD, not only increases the throughput of data but also dramatically reduces the cost of sequencing [9] . Although SNP detection methods for conventional sequencing technologies are well developed, new SNP detection methods for NGS technologies are still lacking. Several methods have been developed for SNP calling from NGS data, and the performances of these SNP calling programs have been evaluated [10] . For example, the SNP calling method by Morin et al. [11] used a proportion of bases that matched the reference. However, this method used an arbitrary threshold and did not provide confidence estimates for the predicted results. Other methods such as MAQ [12] and SOAPsnp [13] , [14] are based on Bayesian-based posterior probabilities, and SNVmix [15] uses a mixed binomial model to discover SNPs, giving a confidence score for each SNP called. These methods perform better for loci with high sequence depths, but their accuracy decreases for sequence depths lower than 10. Other SNP callers used in NGS analysis are integrated into pipelines or are structured into software libraries, such as Bcftools [16] in samtools and UnifiedGenotyper in GATK [17] . Both of these tools use Bayesian likelihood to infer the posterior probability of a locus being a SNP and to call the genotype. Furthermore, both methods can use pooled data to improve the accuracy of the SNP calling. A recent software tool [18] was developed for SNP calling of lower sequencing depths. However, the SNP filtering parameters were manually defined and the program accepted inputs from only the Solexa platform. This software performed better when known SNPs of the target genome were available. We have designed a fast and accurate SNP detection (FaSD) program that uses a binomial distribution-based algorithm and a mutation probability to detect SNPs from NGS data. We compared our method with existing software using both cancer and normal tissue data from The Cancer Genome Atlas (TCGA) [19] and trios data from 1,000 Genomes Project [20] . Using SNP arrays and high-depth sequencing data as benchmarks, we found that our method had higher SNP calling accuracy compared with other methods, especially with low-depth sequencing data. Furthermore, our program completed the SNP calling from 10-fold human genome NGS data (30 gigabases) within four hours on a standard desktop computer compared with the GATK method that takes double the time. Performance evaluation on SNPs covered by arrays To assess the SNP calling quality of the tools, we compared the results from our FaSD method with GATK [17] , SOAPsnp [13] , [14] , MAQ [12] , SNVmix2 ( [15] ) and Bcftools [16] using data sets derived from a Glioblastoma multiforme (GBM) tumour sample and the corresponding blood normal sample from the same individual, which were both sequenced on a Illumina Genome Analyzer II platform. We used genotype calling results from both Affymetrix and Illumina SNP arrays as gold standards, which were obtained from the same samples. Because of the poor accuracy of SNP calling for data with very low sequencing depths [12] , [13] , we included only the loci that were covered by at least four reads. We compared the genotype concordances [17] ( Supplementary Table S1 ) among the SNP calling tools and the two SNP arrays for both normal and tumour data sets. 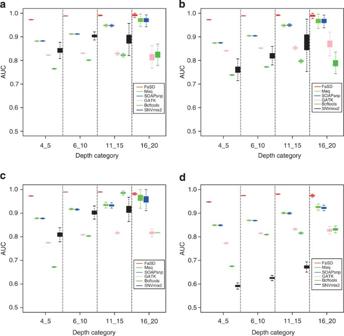Figure 1: Box plots of the AUC of each program based on 1,000 times bootstrap. The average depth of this data set was 10 × . (a) The normal data set with Affymetrix SNP array as the benchmark, (b) normal data set with Illumina SNP array as the benchmark, (c) tumour data set with Affymetrix SNP array as the benchmark and (d) tumour data set with Illumina SNP array as the benchmark. The average sequencing depth in both normal and tumour data sets was 10 × . The number of loci located in the 16_20 category was less than the number of loci located in the other categories. This explains why some tools in 16_20 category showed a small decrease in the AUC with a corresponding slight increase in the standard deviation compared with the other categories. Looking at the normal data set with either Bowtie ( Table 1 ) or BWA ( Supplementary Table S2 ) as the aligner, the genotypes called by both Affymetrix SNP array 6.0 and Illumina humanhap550 genotyping beadchip array were very similar with concordance rates of more than 0.95 (0.997 for bowtie and 0.957 for BWA). SOAPsnp and MAQ, both developed by the Beijing Genome Institute in Shenzhen, China, also showed high concordances of 0.997 with either Bowtie or BWA as the aligner. The genotypes called by GATK and Bcftools were very similar when using Bowtie as the aligner giving a concordance of 0.979. The concordance drops to 0.924 when BWA was used as the aligner, but this value was still high compared with other genotype calling methods. By comparing the results from the SNP calling programs with those from the two arrays used as our gold standards, we found that FaSD and Bcftools were the best methods. FaSD was better than Bcftools when Illumina array was used as the benchmark ( Table 1 and Supplementary Table S2 ), as shown by a concordance of 0.882 for FaSD vs. 0.865 for Bcftools when aligned by Bowtie, and 0.833 vs. 0.674 when aligned by BWA. We also evaluated the performance of these methods on the tumour data set, because tumour tissues are highly heterogeneous compared with normal tissue. With either Bowtie or BWA as the aligner, FaSD showed a higher concordance of about 3–5% with benchmarks in the tumour tissue compared with normal tissue ( Table 1 and Supplementary Table S2 ). Similar concordance increases were observed in Bcftools with both Bowtie and BWA, but this was not the case for others. In contrast, MAQ and SOAPsnp showed a slight drop in concordance for tumour tissue compared with normal tissue. Table 1 The genotype concordance rates among distinct SNP callers with Bowtie as the aligner. Full size table The area under the curve (AUC) of a receiver operating characteristic (ROC) curve is widely used as a measure of the overall classification performance of a program without needing to consider the specific cutoffs. We independently evaluated the performances by comparing the AUCs of different programs using both normal and tumour data sets. Because the sequencing depth has a large impact on SNP calling quality, we separated all the data sets into four sub-data sets according to the sequencing depth of each position. The subsets were named 4_5, 6_10, 11_15 and 16_20, which corresponded to sequence depths of 4–5, 6–10, 11–15 and 16–20, respectively. As shown in Supplementary Tables S3 and S4 , FaSD had the largest AUC compared with the other tools for all the sub-data sets of both the tumour and normal data sets, regardless of the array platform used as the benchmark. We further tested the performances by the stability of AUCs (bootstrapped 1,000 times), and the result confirmed that FaSD significantly outperformed the other methods, especially in low coverage categories ( Fig. 1 , one tail unpaired Wilcox test P <2.2e−16 for each depth category, in both GBM tumour and normal data sets, benchmarked by either Illumina or Affymetrix array). Figure 1: Box plots of the AUC of each program based on 1,000 times bootstrap. The average depth of this data set was 10 × . ( a ) The normal data set with Affymetrix SNP array as the benchmark, ( b ) normal data set with Illumina SNP array as the benchmark, ( c ) tumour data set with Affymetrix SNP array as the benchmark and ( d ) tumour data set with Illumina SNP array as the benchmark. The average sequencing depth in both normal and tumour data sets was 10 × . The number of loci located in the 16_20 category was less than the number of loci located in the other categories. This explains why some tools in 16_20 category showed a small decrease in the AUC with a corresponding slight increase in the standard deviation compared with the other categories. Full size image We compared the results from FaSD, GATK, Bcftools and MAQ on both normal and tumour data sets. For the tumour samples using Affymetrix SNP array as the benchmark, SNPs were divided into several groups: SNPs detected by a single tool, two tools, three tools and by all four tools ( Fig. 2 ). For a SNP called by FaSD and by either Bcftools or GATK, over 99.7% could be confirmed by the Affymetrix array. However, if a SNP was called by both Bcftools and GATK, but not by FaSD, only 46.2% could be confirmed by the Affymetrix array. We further looked at the SNPs that were called uniquely by each tool: 63.3% of SNPs detected by only FaSD could be confirmed by the Affymetrix array, whereas the number was 43.3% for GATK, 35.9% for Bcftools and 2.0% for MAQ. MAQ made the largest number of SNP calls, but the accuracy was the lowest for uniquely called SNPs. We analysed the normal data set and found similar results ( Supplementary Fig. S1 ). 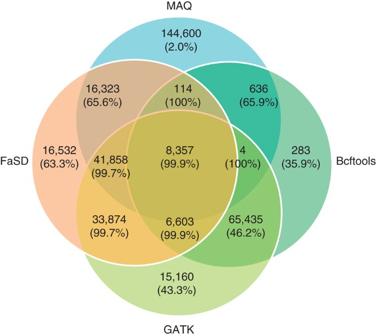Figure 2: The Venn diagram of SNPs detected by different tools. The number in each cell is the number of SNPs in the corresponding category. The percentage under the number is the proportion of SNPs that were confirmed by the Affymetrix SNP array. The FaSD, GATK, Bcftools and MAQ called 123661, 171291, 81432 and 211892 SNPs in total, respectively. The average depth of this data set was 10 × . The figure is based on the tumour data set and Bowtie was used as aligner, and statistics are based on the loci genotyped by the Affymetrix SNP array. Figure 2: The Venn diagram of SNPs detected by different tools. The number in each cell is the number of SNPs in the corresponding category. The percentage under the number is the proportion of SNPs that were confirmed by the Affymetrix SNP array. The FaSD, GATK, Bcftools and MAQ called 123661, 171291, 81432 and 211892 SNPs in total, respectively. The average depth of this data set was 10 × . The figure is based on the tumour data set and Bowtie was used as aligner, and statistics are based on the loci genotyped by the Affymetrix SNP array. Full size image Performance evaluation on SNPs not covered by arrays Both Illumina and Affymetrix SNP arrays contain less than one-tenth of the total number of current SNPs in the human genome, so evaluations based on the SNP arrays will be biased for common SNPs selected by these platforms. To avoid this bias, we evaluated the performance of the tools using high coverage multi-source-merged sequencing data (chromosomes 21 and 22 from a Yoruba with average 35-fold whole genome coverage). Because this data set has high sequence depth and MAQ has been proven to have high SNP calling accuracy for high sequence depth data [12] , we used the results of MAQ SNP calling (named High_MAQ) on this data set as our benchmark. We randomly sampled 10% of reads four times to form four sub-data sets. FaSD, MAQ, SOAPsnp, GATK and Bcftools were then used to call SNPs on these sub-data sets and their results were compared with the benchmark. The majority of loci (>99.5%) in the human genome have the genotype of AA, whose inclusion could overwhelm any differences, that is, the overall genotype concordance won’t differ much among the various caller methods. Therefore, we used non-reference concordances to assess the quality of SNP calling by excluding the concordant AA genotypes ( Supplementary Table S1 ). As shown in Table 2 , with default cutoffs, FaSD called 69,768 SNPs in chromosome 21 and 78,240 SNPs in chromosome 22. The numbers are close to the SNPs called by the benchmark, which were 78,679 and 68,017, respectively. SOAPsnp and MAQ called 25–40% more SNPs than the benchmark, whereas Bcftools and GATK called 40–50% less SNPs than the benchmark. To call a similar number of SNPs as Bcftools and GATK, we adjusted FaSD’s cutoff from the default 3.2 to 5.0, which reduced numbers of SNPs called in chromosomes 21 and 22 to 45,845 and 45,211, respectively. We then compared the non-reference concordances of FaSD at this cutoff with the other tools and with the benchmark. 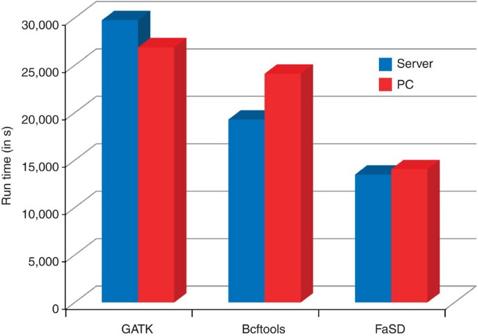Figure 3: Run time on both server and standard personal computer. The average depth of this tumour data set was 10 × (30 gigabases). Bowtie is applied as aligner. For chromosome 21, FaSD had the highest non-reference concordance with the benchmark ( Table 3 ). Consistent with our previous evaluation, the performance of SOAPsnp was almost the same as MAQ [10] . The non-reference concordances of both GATK and Bcftools with the benchmark were also around 0.4, which was close to that of FaSD. For chromosome 22, GATK had the best non-reference concordance with the benchmark. However, the non-reference concordances of both FaSD and Bcftools were only around 0.5% and 2.5% lower than GATK, respectively ( Supplementary Table S5 ). Table 2 Number of reported SNPs in each method for chromosomes 21 and 22. Full size table Table 3 The non-reference concordances for chromosome 21. Full size table Performance evaluation on pooled data The detection of rare variants is important because common genetic variants can explain only a small proportion of heritability [21] . However, rare variants have low minor allele frequencies and are very hard to separate from genotype errors [22] . Pooled data from multiple individuals can improve the discovery of rare variants. Both GATK and Bcftools have the function to utilize pooled data. Therefore, we compared the performance of FaSD on pooled samples with the performance of both GATK and Bcftools. The pooled samples are composed of low coverage (~4 × ) whole genome sequencing data of 40 CEU (Utah residents with ancestry from Northern and Western Europe) individuals from pilot 1 of 1,000 Genomes Project. Sequencing data on chromosome 21 of three CEU individuals in one trio were picked as the evaluation objects. MAQ calling results of corresponding high coverage data (30 × ) from pilot 2 of 1,000 Genomes Project were used as the gold standard. As expected, the calling results on the individual’s low coverage 4 × data had limited SNPs discovery. 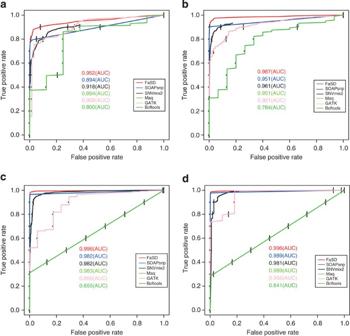Figure 4: The performance on the OV data set sequenced from the SOLiD sequencing platform. (a) The AUC on the 4_5 coverage subset, (b) the AUC on the 6_10 coverage subset, (c) the AUC on the 11_15 coverage subset and (d) the AUC on the 16_20 coverage subset. The average depth of this data set was 6 × . Even using FaSD as the caller, we could not exceed the non-reference concordance of 0.6 ( Table 4 and Supplementary Tables S6 and S7 ). Using a multi-sample SNPs calling function to genotype multiple samples simultaneously from aggregated 40-sample data, GATK and Bcftools showed at least 20% improvement in terms of the non-reference concordance. FaSD also showed a slight increase in the non-reference concordance because it also incorporated genotype information from the pooled data sets. For all individuals investigated from that trio, FaSD had the best non-reference concordances of 0.557 (NA12878), 0.585 (NA12891) and 0.556 (NA12892) benchmarked by High_MAQ. In the GATK pipeline, imputation [23] , [24] could help to refine and recover genotypes at sites with little or no coverage. Following this recommendation, we used Beagle [25] to impute the 40-sample call set. It should be noted that imputation not only recovered an additional 36% of the non-reference sites for FaSD, 26% for GATK and 3% for Bcftools (average of three individuals, Supplementary Table S8 ), but also improved the non-reference concordance from an average of 0.566 to an average of 0.706 for FaSD, from 0.477 to 0.632 for GATK and from 0.514 to 0.590 for Bcftools (average of three individuals, Supplementary Tables S9–11 ). Table 4 The non-reference concordances for chromosome 21 in individual call set and pooled-sample call set of NA12878. Full size table Processing speed The time taken for these tools to process the data is a major bottleneck for NGS data analysis. We compared the running time of FaSD, GATK and Bcftools for SNP calling on a standard 10-fold tumour genome (total 30 gigabases) NGS data. All three programs were tested on a server (based on a 2.13-GHz Intel Xeon Processor E5506 CPU with 4 MB cache, 32 GB memory and 4 TB storage) and on a standard personal computer (running a 2.66-GHz Intel Core2 Quad Processor Q9400 CPU with 6 MB cache, 6 GB memory and 1 TB storage). On the server using only a single core, GATK took 29,757 s to finish the job and Bcftools took 19,286 s, whereas FaSD took only 13,484 s, which was 120% faster than GATK and 43% faster than Bcftools ( Fig. 3 ). On the personal computer, FaSD finished the job in 14,042 s, which was 92% faster than GATK and 72% faster than Bcftools. Figure 3: Run time on both server and standard personal computer. The average depth of this tumour data set was 10 × (30 gigabases). Bowtie is applied as aligner. Full size image Our FaSD method could rapidly call SNPs after the NGS data are aligned to the reference genome. FaSD uses a single score (FaSD_score) to determine the loci’s genotype. For all the experiments, we used a default cutoff of 3.2 for separating AA and AB, and a cutoff of 15.8 for separating AB and BB. Users can adjust these cutoffs in our program to obtain different numbers of SNPs depending on their purpose. As shown in Supplementary Table S12 , a higher cutoff will result in less SNPs being reported, and vice versa. If the default cutoff of 3.2 is applied, the false positive rate and true positive rate are 0.0011 and 0.83 in the normal data set and 0.0015 and 0.82 for the tumour data set, respectively. To assess the AUC of each SNP caller, we assigned a SNP locus as class 1, and a non-SNP locus as class 0. The 0/1 ratio is the ratio between the numbers of loci in class 0 and class 1. The loci were determined to be truly class 0 or class 1 based on the gold standard used. An imbalanced data set could reduce the classification performance and make the classifications deviate to the prevalent class [26] , [27] . The 0/1 ratios of both the normal data set and tumour data set were close to 1 ( Supplementary Table S13 ), indicating little classification bias in our array-based data sets. Our FaSD algorithm is comprised of two parts, the alternative_score and the mutation probability (equations 1 and 2 in the methods section). The mutation probability model has been used in many other SNP detection programs. We report here for the first time the use of our unique alternative_score model. To assess the contributions of these two models to the overall performance of the FaSD method, we evaluated the AUCs separately and in combination from the normal data set benchmarked by the Affymetrix array. In the 4_5 depth category ( Table 5 ), the combined model had an AUC of 0.973, which decreased by 0.033 to 0.940 when only the mutation probability model was used but only decreased by 0.003 to 0.970 when only the alternative_score model was used, indicating the alternative_score model contributed about 90% to FaSD’s performance. At high depth, the AUC decreased by 0.009 using only the mutation probability model but decreased by 0.001 using only the alternative_score model, indicating the alternative_score contributed about 70–80% to FaSD’s performance. Similar results were obtained when the two components were evaluated using the Illumina array ( Table 5 ). Table 5 AUC of different parts of FaSD on the normal data set. Full size table To assess the effects of different aligners on FaSD’s performance, we used BWA as alternative aligner for the tumour and normal data set (BWA is the recommended aligner for GATK). On the basis of concordance, we showed that FaSD was the superior method ( Supplementary Table S2 ). Although with BWA the AUC of GATK increases by about 10% in each sub-category, FaSD still has the largest AUCs ( Supplementary Table S14 ), indicating FaSD’s superior performance regardless of the aligner. We then assessed the effects of the sequencing platform on FaSD’s performance. We used the six tools to call SNPs from data sequenced using ABI-SOLiD sequencing platform. With the Affymetrix SNP array as the gold standard, FaSD outperforms all the other programs using the corresponding Serous Cystadenocarcinoma (OV) data set (One tail paired Wilcoxon test P -value <2.2e-16 in each depth category, Fig. 4 and Supplementary Fig. S2 ). This result confirmed that FaSD SNP calling is reliable even for data from different sequencing platforms. Figure 4: The performance on the OV data set sequenced from the SOLiD sequencing platform. ( a ) The AUC on the 4_5 coverage subset, ( b ) the AUC on the 6_10 coverage subset, ( c ) the AUC on the 11_15 coverage subset and ( d ) the AUC on the 16_20 coverage subset. The average depth of this data set was 6 × . Full size image The developers of GATK proposed a unified analytic framework that included realigning the sequences before SNP calling to reduce the effects of inaccurate base quality scores and mapping errors [23] . We adopted this framework for locally realigning regions around indels and for recalibrating the base quality score to check how the pre-process affected the SNP calling quality. Realignment had significant effects on GATK’s performance, particularly when using the Affymetrix array as the gold standard. Realignment caused GATK’s concordance rates with the Affymetrix array to increase from 0.839 to 0.912 for normal tissue and increase from 0.875 to 0.930 for tumour tissue. Changes in FaSD performance resulted in a moderate concordance increase from 0.891 to 0.922 for normal tissue and an insignificant increase from 0.926 to 0.929 for tumour tissue ( Tables 1 and 6 ). On the other hand, realignment with Illumina Array as the gold standard had an overall negative effect. After realignment, the concordance rates between Illumina and Affymetrix arrays dropped from 0.997 to 0.949 for normal and from 0.996 to 0.942 for tumour tissues. The effects were most pronounced for Bcftools, dropping from 0.865 to 0.735 for normal and from 0.898 to 0.734 for tumour tissues. For FaSD, changes were 0.882 to 0.864 for normal and 0.927 to 0.867 for tumour tissues. Both MAQ and SOAPsnp had better concordance rates with the Illumina array after realignment. For MAQ, changes were 0.397 to 0.439 for normal and 0.401 to 0.469 for tumour tissues, and for SOAPsnp, changes were 0.417 to 0.439 for normal and 0.409 to 0.472 for tumour tissues ( Tables 1 and 6 ). We further evaluated the AUC of the different tools after realignment. We found that FaSD performed better than the other tools regardless of whether the data was pre-processed or not, or whether the Affymetrix or Illumina array benchmarks were used ( Supplementary Tables S15–18 ). Table 6 The concordance rates after realignment among distinct SNP callers. Full size table We evaluated the performance of the different tools using the three criteria of concordance rate, AUC and non-reference concordance rate. These criteria were applied in different situations ( Supplementary Table S1 ). When one of the two callers is used as the benchmark, the concordance rate is used to measure the proportion of correctly called AA, AB and BB genotypes in the results. The SNP caller must use a specific cutoff for genotype calls, so the concordance will only be valid under this cutoff. In contrast, AUC measures the overall performance of two classification groups, AA and non-AA (non-SNP and SNP). It is a comprehensive measurement because it is not limited to a specific cutoff, but it does not distinguish between AB and BB. Therefore, the concordance and AUC measurements may not always be consistent. For example, Bcftools has high concordance rates ( Table 1 and Supplementary Table S2 ) but poor AUC ( Supplementary Tables S3 and S4 ). When a program is applied on genome-wide data, the SNP calling result will be highly unbalanced because the chance of calling a SNP is less than 1% (predominately AA). Under this situation, the non-reference concordance rate is more appropriate than concordance rate for performance assessment, because it focus on measuring the quality of called AB and BB genotypes. FaSD can be used as good complementary program to either GATK or Bcftools. The accuracy rate for SNPs called by both FaSD and Bcftools was the highest at 99.9% ( Fig. 2 ). For SNPs called by both FaSD and GATK, the rate was also high at 99.7%. In contrast, the accuracy is far less for SNPs called by any other two programs. For example, SNPs called by both FaSD and MAQ (but not by others) had an accuracy rate of 65.6%, and for GATK and Bcftools the accuracy was 46.2%. SNPs called individually by FaSD, GATK, Bcftools and MAQ had accuracies of 63.3%, 43.3%, 35.9% and 2.0%, respectively. We further investigated SNP loci called uniquely by FaSD and confirmed by both Affymetrix and Illumina SNP arrays (some examples are shown in Supplementary Figs S3–S5 ). In general, FaSD made accurate SNP calls even at loci with low-depth reads, with intermediate sequencing quality, and at the two ends of the read, compared with other programs that failed to make SNP calls. In summary, we recommend using both FaSD with either GATK or Bcftools for SNP calls. If the user requires a larger number of SNP calls, we suggest using FaSD on its own or FaSD and MAQ combined. The next best option would be to use GATK on its own or GATK and Bcftools combined. The FaSD program was implemented in C ++ , which can easily be compiled to run on all platforms. Once the result of alignment is obtained, our model is able to detect SNP sites with high speed based on the pileup files. The compiled programs for Linux or Windows and demonstration data can be downloaded freely at http://jjwanglab.org/FaSD . Data sets We used NGS data from both a blood-derived normal sample and GBM tumour sample sequenced in the TCGA project. The reads (Sequence Read Archive (SRA) accession code: SRX006325 ) of the blood-derived normal sample (TCGA accession code: TCGA-06-0188-10B-01D-0373-08) were from a male with untreated GBM (TCGA accession code: TCGA-06-0188). The reads (SRX006310) of the GBM tumour sample were from primary tumour tissue (TCGA-06-0188-01A-01D-0373-08) from the same male with untreated GBM (TCGA-06-0188) [19] . Both the samples were sequenced on the Illumina Genome Analyzer II platform: the normal sample was prepared by 2 × 76 bp paired-end library construction (Solexa-8304) and the GBM sample was prepared by 2 × 76 bp paired-end library construction (Solexa-8303). To evaluate NGS data from the SOLiD platform, reads (SRX015368) from the primary tumour tissue (TCGA-13-0720-01A-01D-0445-10) of a female OV patient (TCGA-13-0720) were used (~6-fold). The sequences, all in fastq format (csfastq for SOLiD), were extracted from the NCBI database of genotype and phenotype (dbGap) using the SRA toolkit. The raw data obtained using SRA was not filtered or modified (besides trimming). We merged the results from several runs to reach 30 gigabases at 10 × coverage for each data set. These data sets were also genotyped using Illumina humanhap550 genotyping beadchip array and Affymetrix genome-wide human SNP array 6.0. The genotype data were downloaded from TCGA portal and used as our gold standards. To test the SNP callers’ performance without using SNP arrays as the benchmark, we used data from one Yoruba individual (1,000 genomes accession code: NA19240) with high coverage MAQ alignment data of chromosome 21(39 × ) and 22(40 × ) generated by the pilot 2 phase of 1,000 Genomes Project [28] . To compare the performance of FaSD on pooled samples with the performance of GATK and Bcftools, we used the publically available sequencing data from 40 CEU individuals in the pilot 1 phase of 1,000 Genomes Project. All 40 individuals were sequenced to ~4 × coverage genome-wide on a variety of platforms and from a variety of sequencing centres [29] . Sequencing data on chromosome 21 of a CEU trio (NA12878, NA12891 and NA12892) out of the 40 individuals was chosen as our evaluation subjects. This trio was also sequenced to ~30 × coverage genome-wide in the pilot 2 phase of 1,000 Genomes Project. We used MAQ’s SNPs calling result on chromosome 21 of this high-depth trio, NA12878 (37 × , rounded sequencing depth of chromosome 21), NA12891 (36 × , rounded) and NA12892 (30 × , rounded) as the evaluation benchmark. The FaSD model After obtaining alignments from pileup file, we used FaSD to call SNPs for each aligned position. A FaSD_score was used to measure the polymorphism probability that a certain locus is a SNP location and to determine its corresponding genotype. If the FaSD_score was greater than the cutoff score, we called the locus a SNP and gave its corresponding genotype. The FaSD_score was calculated using the alternative_score and the geometric mean of a mutation probability of reads (equation 1): The alternative_score was calculated according to equation 2. The is the probability of getting a read genotype when the reference allele is known [30] . At each position, there could be three possible genotypes: AA, AB and BB. AA is homozygous and matches the reference allele, AB is heterozygous and BB is homozygous but does not match the reference allele. For positions with depth N , n reads will match the reference and the other N − n reads will not match the reference. We assumed that the number of reads matching and not matching the reference will follow binomial distributions. We then calculated the probability of the observed read frequency for each of the three possible genotypes. If the genotype is AA, then the probability of not matching the reference should be very low (to be consistent with the error rate in the mutation probability formula we set this to 0.001), and thus the probability of matching the reference should be very high (we set this to be 1–0.001=0.999). If the genotype is AB, the probability of matching the reference and non-reference should be equal (both set to 0.500). Similarly, if the genotype is BB, the probability of matching the reference should be 0.001 and of matching the non-reference should be 0.999 (equation 2). We then used the probability mass function of binomial distributions to calculate the joint probability of all N reads. We then compared the joint probabilities from all three possible genotypes. The genotype with the highest probability was selected and the alternative_score was assigned (equation 2). The three different binomial distributions corresponding to AA, AB and BB were assigned the P parameter 0.001, 0.500 and 0.999, respectively. We then checked whether these parameters fitted our data. Taking into account the possible flaws in the sequencing, alignment or construction of the data sets, the parameters for the three binomial distributions appeared to be acceptable. The assigned alternative_score of 0, 1 and 2 represents the number of loci that are different from the reference allele for two allele loci. Positions with genotype AB or BB are considered as SNP locations. N is the depth of the reads, and m is the occurrence of reference allele at the position. We added a pseudo_score to avoid an alternative_score of 0. By default, we set the pseudo_score to 0.01. The alternative_score depends on which one of the three possible genotypes/models (reference homozygote, non-reference homozygote, and heterozygote) explain the data the best. For example, if the locus has a total of five reads, with three Gs and two Cs, and the corresponding reference is G: the probability of getting the above reads with the reference homozygote model is ; the probability for the heterozygote model is ; the probability for the non-reference homozygote model is . We choose the heterozygote model because it has the highest probability of 0.31, and we assign an alternative_score=1+0.01=1.01. Using equation 1, we obtain a FaSD_score of 5.07, which is between our default cutoffs of 3.2 and 15.8, so we assign heterozygous genotype GC to this locus. The estimated SNP rate between two distinct human haploid chromosomes has been reported to be close to 0.001 ( [30] ), and transitions are almost four times more frequent than transversions among substitutions [31] . The different frequencies of transitions and transversions mean they would have different contributions to the SNP calling. To discriminate these contributions, we integrated a for each read into our final FaSD_score. We calculated the SNP rate and transition/transversion ratio in our GBM tumour and normal data sets, and found similar ratios (data not shown). Therefore, we used the above reported values to calculate ( Supplementary Table S19 ). For each read, we compared the base at current loci with the reference allele to obtain a . From this table, we calculated the geometric mean of the mutation probability using equation 1. We incorporated the effects of transitions and transversions into our FaSD model. The average of log-odd of all the N reads was obtained, and the product of this value with the alternative_score was combined to form a FaSD_score, which was used to call SNPs. The higher the FaSD_score, the more likely a site is a SNP position. The default cutoffs of FaSD are determined mathematically. Because different types of errors such as sequencing or mapping errors during NGS could raise the FaSD_score of a non-SNP site, we suggest the use of a cutoff value higher than the default to remove false positives, especially with low quality sequencing data. A user interface for setting the user-specific cutoff has been implemented in our FaSD program. The model has the ability to handle both the individual data sets and the pooled data sets. Performance evaluation using SNP arrays We used Illumina and Affymetrix SNP arrays as gold standards to evaluate the performance of FaSD and other tools. We excluded all sites whose depths were lower than 4. The quality score is absent for the Illumina HumanHap550 Genotyping BeadChip data, so we accepted all the genotype entries. The Affymetrix genome-wide human SNP array 6.0 provides confidence scores for genotype quality using the Birdseed algorithm. Here, we chose the high-quality SNP probes as our test data set by removing the probes with confidence scores above 0.018. For SOAPsnp and MAQ, we assigned the Phred-scaled probability that the genotype is identical to the reference, the so called ‘SNP quality’ as the predictor. There are several possibilities for the called genotypes: the reference homozygote, the non-reference homozygote, heterozygote and others. For the ROC curve and AUC calculations, we assigned the reference homozygote genotype as 0, and all other genotypes as 1. SNVmix2 outputs three genotypes, namely homozygous to reference (AA), heterozygous genotype (AB) and homozygous to the non-reference (BB). We considered AB and BB genotypes as a SNP, we added the probabilities of these two genotypes (AB and BB) together to get the ‘SNP probability’ as the predicator. The GATK’s UnifiedGenotyper and Bcftools generate SNP calls in the VCF format; the QUAL column is the ‘SNP quality’ and can be used as our predicator. For all callers mentioned above, the different values of predictor were used to draw the ROC curve, whereas the FaSD_score was used for FaSD. To test the stability of each software, we performed 1,000 times’ bootstrap and obtained 1,000 AUC for each software. We then used Wilcoxon test to determine whether FaSD performed better than the other tools. The genotype concordance and non-reference concordance To measure the reliability of the different software/platforms for genotypes called from all SNPs (not limited to SNPs in Illumina and Affymetrix arrays), we determined genotype concordances among tools. Before the calculation of concordance, we restricted the tested loci to be the loci which has been genotyped in benchmark and whose depth were higher than 3 in the test alignment file to facilitate the reliability of the concordance result. Because GATK and Bcftools only report non-reference sites, we assigned genotype AA, the reference homozygous, to the loci which are not listed in SNP calling result of the above two tools. The non-reference concordance is measured in the similar way but excludes the concordant AA genotype because they are usually huge in number and easily detectable, but will greatly influence the measurement. How to cite this article: Xu, F. et al. A fast and accurate SNP detection algorithm for next-generation sequencing data. Nat. Commun. 3:1258 doi: 10.1038/ncomms2256 (2012).